Exosomes as Hedgehog carriers in cytoneme-mediated transport and secretion The Hedgehog signalling pathway is crucial for development, adult stem cell maintenance, cell migration and axon guidance in a wide range of organisms. During development, the Hh morphogen directs tissue patterning according to a concentration gradient. Lipid modifications on Hh are needed to achieve graded distribution, leading to debate about how Hh is transported to target cells despite being membrane-tethered. Cytonemes in the region of Hh signalling have been shown to be essential for gradient formation, but the carrier of the morphogen is yet to be defined. Here we show that Hh and its co-receptor Ihog are in exovesicles transported via cytonemes. These exovesicles present protein markers and other features of exosomes. Moreover, the cell machinery for exosome formation is necessary for normal Hh secretion and graded signalling. We propose Hh transport via exosomes along cytonemes as a significant mechanism for the restricted distribution of a lipid-modified morphogen. The Hh molecule acts as a morphogen to regulate growth and cell fate specification at a distance. In different systems, Hh is secreted from a restricted group of cells and distributed in a concentration-dependent manner according to distance from the source, resulting in differential activation of target genes [1] . Thus, Hh production, release, transport and reception must be kept under strict spatial and temporal control to accomplish an activity gradient. Hh gradient formation mechanisms have been studied extensively in the Drosophila wing imaginal disc comprising two cell populations with different adhesion affinities dividing the field into a posterior (P) and an anterior (A) compartment. The P compartment cells produce Hh, which moves across the A/P compartment border, decreasing in concentration as it spreads away from the border to the A compartment (scheme in Fig.1a ). Hh is post-translationally modified by the addition of cholesterol [2] and palmitic acid [3] , which promote Hh association to lipid membranes but are essential for its restricted spreading [4] , raising the question of how its actual secretion and transfer are achieved. In both the wing disc and the abdominal epidermis of Drosophil a, specialized filopodia called cytonemes [5] are crucial for establishment of the Hh gradient [6] . Cytonemes are easily visualized by confocal microscope in the basal part of the wing disc epithelium by expressing the Hh co-receptor Interference hedgehog (Ihog) [6] , [7] , [8] , which also labels punctate structures [8] with a size of 0.1–0.6 μm; some of them seem to exceed the cytoneme diameter, suggesting they could be extracellular vesicles (EVs) [6] . In the chicken limb bud, particles containing SonicHh (SHh) and CDO (vertebrate homologue of Ihog) have also been shown to travel along filopodia-like extensions within the field of SHh signalling [9] . Here we characterize these structures and their association with Hh, determining the role of EVs in Hh distribution and gradient formation. 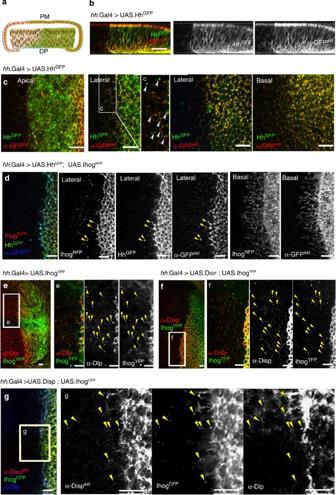Figure 1: Hh and key signalling components are present in EVs and cytonemes. (a) Schematic representation of a cross-section of the wing disc showing the expression of Hh in both epithelia; disc proper (DP) and peripodial membrane. (b) Transverse section of ahh.Gal4>UAS.Hh-GFP wing disc which has beenex vivostained with anti-GFP antibody for 1 h at low temperature to avoid Hh-GFP internalization. Note the co-localization of Hh-GFP and externalized GFP (red) mainly at the basolateral part of the disc epithelium (bottom of image). (c) Confocal sections of a similarhh.Gal4>UAS.Hh-GFP wing discex vivostained with anti-GFP antibody. Note that the co-localization of green and red (externalized Hh) is increased in more basolateral sections. The internalized Hh-GFP at the A compartment is in green (white arrow heads). Note also that in the most basal section Hh puncta appear to be aligned in a ‘beads on a string’ arrangement, suggesting they associate to cytonemes (see also ref.6). (d)Ex vivostaining using an anti-GFP antibody in a UAS.Hh-GFP/UAS.Ihog-RFP;hh.Gal4/tubGal80tswing disc after 24 h at the restrictive temperature. Note the co-localization between Hh and Ihog (arrow heads) in the A compartment and also the presence of externalized Hh at the cellular extensions marked by the Ihog protein. (e) Dlp expression in a tubGal80ts; UAS.Ihoh-YFP/hh.Gal4 wing disc for 24 h. (e) Insets ineshowing the co-localization of puncta of Ihog and Dlp (arrow heads) in the A compartment. (f) Ectopic expression of UAS-Ihog-YFP and UAS-Disp using thehh.Gal4; tubGal80tssystem for 24 h. (f) Insets infshow the co-localization of puncta of both proteins (arrow heads) in the A compartment. (g)Ex vivostaining using an anti-Disp antibody in a UAS-Disp/UAS-iHo-CFP;hh.Gal4/tubGal80tswing disc after 24 h at the restrictive temperature. Note the co-localization of Disp, Dlp and Ihog in the A compartment cells (arrow heads) (insets g). Scale bars,10 μm. Figure 1: Hh and key signalling components are present in EVs and cytonemes. ( a ) Schematic representation of a cross-section of the wing disc showing the expression of Hh in both epithelia; disc proper (DP) and peripodial membrane. ( b ) Transverse section of a hh .Gal4>UAS.Hh-GFP wing disc which has been ex vivo stained with anti-GFP antibody for 1 h at low temperature to avoid Hh-GFP internalization. Note the co-localization of Hh-GFP and externalized GFP (red) mainly at the basolateral part of the disc epithelium (bottom of image). ( c ) Confocal sections of a similar hh .Gal4>UAS.Hh-GFP wing disc ex vivo stained with anti-GFP antibody. Note that the co-localization of green and red (externalized Hh) is increased in more basolateral sections. The internalized Hh-GFP at the A compartment is in green (white arrow heads). Note also that in the most basal section Hh puncta appear to be aligned in a ‘beads on a string’ arrangement, suggesting they associate to cytonemes (see also ref. 6 ). ( d ) Ex vivo staining using an anti-GFP antibody in a UAS.Hh-GFP/UAS.Ihog-RFP; hh. Gal4/tubGal80 ts wing disc after 24 h at the restrictive temperature. Note the co-localization between Hh and Ihog (arrow heads) in the A compartment and also the presence of externalized Hh at the cellular extensions marked by the Ihog protein. ( e ) Dlp expression in a tubGal80 ts ; UAS.Ihoh-YFP/ hh. Gal4 wing disc for 24 h. (e) Insets in e showing the co-localization of puncta of Ihog and Dlp (arrow heads) in the A compartment. ( f ) Ectopic expression of UAS-Ihog-YFP and UAS-Disp using the hh.Gal4 ; tubGal80 ts system for 24 h. (f) Insets in f show the co-localization of puncta of both proteins (arrow heads) in the A compartment. ( g ) Ex vivo staining using an anti-Disp antibody in a UAS-Disp/UAS-iHo-CFP; hh. Gal4/tubGal80 ts wing disc after 24 h at the restrictive temperature. Note the co-localization of Disp, Dlp and Ihog in the A compartment cells (arrow heads) (insets g). Scale bars,10 μm. Full size image Hedgehog is located in EVs that move towards recipient cells In the wing disc, Hh punctate structures (endogenous or ectopically expressed Hh-green fluorescent protein (GFP)) locate at the plasma membrane both apically and basolaterally ( Fig. 1b ), and in both P and A compartment cells near the A/P border [1] ( Fig. 1c ). Importantly, these puncta can be partially labelled by extracellular ex vivo staining with anti-GFP antibody ( Fig. 1b,c ), indicating the presence and the extracellular localization of Hh on their surface. They are more abundant at the basolateral part of the disc epithelium ( Fig. 1b,c red and yellow puncta), and distinct from cytoplasmic puncta [8] (green puncta in Fig. 1c ). The co-expression of Hh-GFP and Ihog-RFP reveals puncta labelled with both markers in the A compartment, as well as puncta that just contain Hh-GFP probably due to internalization of Hh-GFP vesicles by the receiving cells ( Fig. 1d , see also Supplementary Movie 1 ). Live imaging of Ihog-RFP puncta in the abdomen, where Hh also acts as a morphogen [10] , confirms their presence both laterally as well as basolaterally, similar to Hh ( Supplementary Movie 2 ). Dispatched (Disp) [11] and Dally-like (Dlp) [8] , both essential for Hh release [8] , also co-localize with Ihog-labelled punctate structures and cytonemes ( Fig. 1e–g ). These results indicate that Hh could indeed be transported in EVs together with other pathway components, Ihog, Disp and Dlp, all involved in Hh release. The punctate structures localize to cytonemes in the basal side of the epithelium [6] , and as ex vivo antibody staining marks both Disp and Hh, these proteins might all be at the surface of EVs ( Supplementary Fig. 1G ). To further investigate the EV nature of the puncta, immunolabelling for Hh in wing discs co-expressing Ihog-RFP and the mammalian EV marker CD63 tagged with GFP [12] was performed, revealing a clear co-localization of the three in punctate structures ( Fig. 2a ). This co-localization was also confirmed by live imaging in the abdominal epidermis of pupae co-expressing CD63-GFP and Ihog-RFP ( Fig. 2b and Supplementary Movie 3 ). Furthermore, immunoprecipitation of the GFP-tagged CD63 shows co-immunoprecipitation of Ihog-RFP and endogenous Hh in vivo ( Fig. 2c–e ), supporting the presence of CD63 in the Hh–Ihog complex observed by confocal imaging and strongly advocating the EV nature of the puncta ( Fig. 2a,b ). 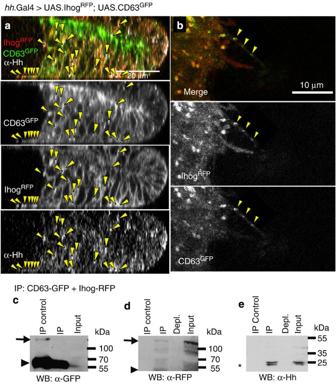Figure 2: Hh and Ihog can complex with the exosome marker CD63in vivo. (a) Lateral view of a reconstructedz-stack of confocal images from a wing disc expressing the exosome marker UAS.CD63-GFP and UAS.Ihog-RFP under the control ofhh.Gal4/tubG80tsafter 24 h at the restrictive temperature and immuno-labelled for Hh. Note the co-localization of Ihog-RFP (red) and the endogenous Hh (grey) with the marker CD63-GFP (arrow heads). Scale bar, 20 μm. (b) Live imaging ofDrosophilaabdomen shows CD63-GFP labelled puncta that co-localizes with puncta also labelled by Ihog-RFP (arrow heads) and that move along the cytoneme (See alsoSupplementary Movie 3). Scale bar, 10 μm. (c–e) Western blots showing co-immunoprecipation of CD63-GFP, Ihog-RFP and endogenous Hh after a GFP-Trap pull down (Chromoteck) from a high-speed supernatant of homogenized larvae expressing CD63-GFP as control and larvae co-expressing CD63-GFP and Ihog-RFP as expermiental. (c) Immunoprecipitation of CD63-GFP shown for both, the IP control and the experimental IP control (arrowhead). (d) Co-immunoprecipitation of Ihog-RFP revealed by anti-RFP in the experimental IP control (arrow) and not present in the IP control. (e) Co-immunoprecipitation of endogenous Hh revealed (after membrane antibody stripping) by anti-Hh in the experimental IP control (asterisk) and not present in the IP control, probably due to an enrichment effect of the co-expression of Ihog-RFP and CD63-GFP. Figure 2: Hh and Ihog can complex with the exosome marker CD63 in vivo . ( a ) Lateral view of a reconstructed z -stack of confocal images from a wing disc expressing the exosome marker UAS.CD63-GFP and UAS.Ihog-RFP under the control of hh. Gal4/tubG80 ts after 24 h at the restrictive temperature and immuno-labelled for Hh. Note the co-localization of Ihog-RFP (red) and the endogenous Hh (grey) with the marker CD63-GFP (arrow heads). Scale bar, 20 μm. ( b ) Live imaging of Drosophila abdomen shows CD63-GFP labelled puncta that co-localizes with puncta also labelled by Ihog-RFP (arrow heads) and that move along the cytoneme (See also Supplementary Movie 3 ). Scale bar, 10 μm. ( c – e ) Western blots showing co-immunoprecipation of CD63-GFP, Ihog-RFP and endogenous Hh after a GFP-Trap pull down (Chromoteck) from a high-speed supernatant of homogenized larvae expressing CD63-GFP as control and larvae co-expressing CD63-GFP and Ihog-RFP as expermiental. ( c ) Immunoprecipitation of CD63-GFP shown for both, the IP control and the experimental IP control (arrowhead). ( d ) Co-immunoprecipitation of Ihog-RFP revealed by anti-RFP in the experimental IP control (arrow) and not present in the IP control. ( e ) Co-immunoprecipitation of endogenous Hh revealed (after membrane antibody stripping) by anti-Hh in the experimental IP control (asterisk) and not present in the IP control, probably due to an enrichment effect of the co-expression of Ihog-RFP and CD63-GFP. Full size image Detailed observation of movies with CD63-GFP marked puncta shows their association with cytonemes in basal regions, where they move along the cytonemes which point from the P towards the A compartment ( Fig. 3a,b and Supplementary Movies 4 and 5 ). Live imaging of cells expressing either the membrane marker CD4-Tomato or Ihog-RFP also shows punctate structures moving along cytonemes ( Fig. 3c,d and Supplementary Movie 6 and 7 , see also ref. 6 ). Interestingly, CD4-Tomato labelling occasionally shows buckling followed by a swelling structure, which might be related to direct shedding of vesicles from the cytoplasmic membrane ( Fig. 3c and Supplementary Movie 6 ), also sporadically observed in puncta labelled with Ihog-RFP ( Fig. 3d and Supplementary Movie 7 ). 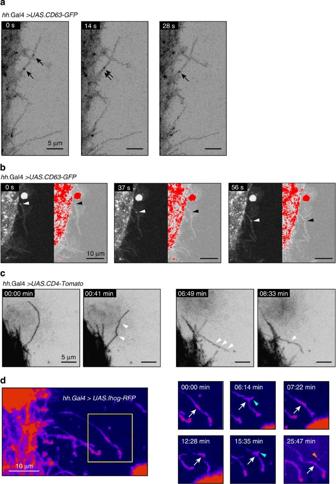Figure 3: Punctate structures move along cytonemesin vivo. (a,b) CD63-GFP labels punctate structures that move along cytonemes. Cells of the P compartment are labelled withhh.Gal4>UAS.CD63-GFP. (a) Individual frames taken fromSupplementary Movie 4. Black arrows indicate puncta. Fluorescence is depicted using an inverted grey lookup table (LUT). (b) Individual frames taken fromSupplementary Movie 5. Arrowheads indicate puncta. Fluorescence is depicted using a grey LUT (left) and a HiLo LUT (right), which highlights the brightest pixels in red. (c) Cytonemes labelled with CD4-Tomato show ‘buckling’ and ‘swelling’. These structures might be related to the shedding of vesicles, which we could observe occasionally (seed). Individual frames taken fromSupplementary Movie 6. Cells of the P compartment are labelled withhh.Gal4>UAS.CD4-Tomato. Fluorescence is depicted using an inverted grey lookup table. (d) Occasionally, we observe punctate structures shedding from the cytonemes. Individual frames taken fromSupplementary Movie 7. Cytonemes reaching into the A compartment are labelled withhh.Gal4>UAS.Ihog-RFP and coloured with a fire lookup table. Left panel: overview. Right panels: time sequence of detail indicated in the overview. Note punctate structures, which are located along the cytonemes. One punctum (white arrows) is budding (cyan arrowheads) and finally shedding from the cytoneme (orange arrowhead). Figure 3: Punctate structures move along cytonemes in vivo . ( a , b ) CD63-GFP labels punctate structures that move along cytonemes. Cells of the P compartment are labelled with hh .Gal4 > UAS.CD63-GFP. ( a ) Individual frames taken from Supplementary Movie 4 . Black arrows indicate puncta. Fluorescence is depicted using an inverted grey lookup table (LUT). ( b ) Individual frames taken from Supplementary Movie 5 . Arrowheads indicate puncta. Fluorescence is depicted using a grey LUT (left) and a HiLo LUT (right), which highlights the brightest pixels in red. ( c ) Cytonemes labelled with CD4-Tomato show ‘buckling’ and ‘swelling’. These structures might be related to the shedding of vesicles, which we could observe occasionally (see d ). Individual frames taken from Supplementary Movie 6 . Cells of the P compartment are labelled with hh .Gal4 > UAS.CD4-Tomato. Fluorescence is depicted using an inverted grey lookup table. ( d ) Occasionally, we observe punctate structures shedding from the cytonemes. Individual frames taken from Supplementary Movie 7 . Cytonemes reaching into the A compartment are labelled with hh. Gal4 > UAS.Ihog-RFP and coloured with a fire lookup table. Left panel: overview. Right panels: time sequence of detail indicated in the overview. Note punctate structures, which are located along the cytonemes. One punctum (white arrows) is budding (cyan arrowheads) and finally shedding from the cytoneme (orange arrowhead). Full size image Immuno-EM reveals Hh in MVB/EV and plasma membrane To analyse the distribution of Hh at the ultrastructural level, immunoelectron microscopy (Immuno-EM) was performed on thawed cryosections of wing discs expressing Hh-GFP. Supplementary Fig. 1A–F shows correlative light-electron microscopy of the Hh distribution on ultra-thin cryosections cut orthogonal to the ventral/dorsal axis. Immunofluorescent Hh staining ( Supplementary Fig. 1A ) was detected along the whole apical disc lumen and at the basolateral region of the P compartment. At the EM level, apical Hh signal was found on microvilli membranes ( Supplementary Fig. 1B ), whereas basolateral staining on Hh-producing cells was mainly detected within multivesicular bodies (MVBs) and lysosomes as well as on the basolateral membranes ( Supplementary Fig. 1C–E ). Interestingly, Hh staining was also detected on heterogeneous vesicle-like structures (size ranging from 30 to 200 nm) in basolateral extracellular spaces close to the basal lamina ( Supplementary Fig. 1F,f ). To further explore the extracellular distribution of Hh, wing discs expressing Hh-GFP were labelled ex vivo with an anti-GFP antibody before EM processing. As shown in Fig. 4a,b , thawed cryosections labelled with a dual fluorescent and electron-dense Fab′fragment probe showed apical staining and a basolateral punctate fluorescent pattern at the P compartment, fully consistent with the punctate labelling of external Hh observed at the confocal microscope ( Fig. 1 ). In addition, at the EM level, immunogold staining detected Hh-GFP on apical microvilli membranes (arrows in Fig. 4c, d ) as well as on discrete regions of basolateral membranes (arrows in Fig. 4f,j ), frequently associated with cell-to-cell contacts (arrows in Fig. 4j ). Importantly, significant Hh labelling was detected on clusters of vesicle-like structures at the basolateral extracellular spaces (arrowheads in Fig. 4g,m,n,p ) and some of these vesicles appear also localized in association with cell protrusions (arrowheads in insets Fig. 4 g and m). Finally, immuno-EM confirmed the presence of Hh, Ihog and Disp at MVBs and exovesicles ( Supplementary Fig. 1G–I ) in cryosections of wing discs expressing Ihog-CFP and Disp-YFP, respectively. Altogether, these results support the notion that all these Hh signalling pathway components share the same secretion mechanism in exovesicles at basolateral spaces. 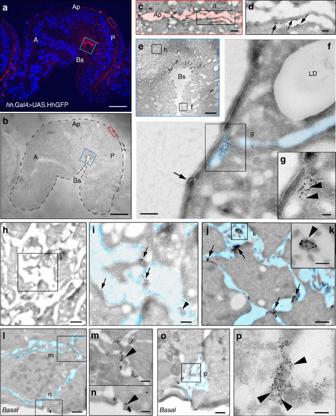Figure 4: Ultrastructural localization of Hh in imaginal discs. Correlative light-electron microscopy of wing discs expressing Hh-GFP. Discs were labelledex vivowith a rabbit anti-GFP antibody and then fixed and processed for cryosectioning. Ultra-thin sections, cut orthogonally to the V/D axis, were incubated with a fluorescent (Alexa594) 1.4-nm nanogold-conjugated anti-rabbit Fab’ probe. Labelled cryosections were first imaged at the fluorescence microscope (a) and then at the transmission electron microscope after silver enhancement of the nanogold signal (b–p). At the light microscopy level (a) fluorescent labelling is detected at apical areas and at basolateral regions of the P compartment. At the EM level, apical immunogold labelling (canddshows the area delimited by a red box inb) decorated microvilli membranes (arrows ind), whereas basolateral signal (f–ishows EM images of the area delimited by a blue box inb, whilej–pshows details of a different disc) is mainly associated with discrete extents of the plasma membrane (arrows inf,i,j) that frequently coincide with cell-to-cell contacts (arrows inj). Also, immunogold labelling is detected in clusters of EV-like structures (arrowheads in g,i,k,m,n,p), some of which are associated with cell protrusions (insets inf(g) andl(m)). A and P compartments as well as apical (Ap) and basolateral (Bs) regions are indicated inaandb. To help the interpretation, apical and basolateral extracellular spaces are depicted in red (c) and blue (f,i–p), respectively.atoicorrespond to the same wing disc, whereasjtopcorrespond to a different specimen. LD, lipid droplet. Scale bars, 25 μm (a,b), 5 μm (e), 500 nm (c,h,j,l,o), 200 nm (d,f,i,k,m,n) and 100 nm (g,p). Figure 4: Ultrastructural localization of Hh in imaginal discs. Correlative light-electron microscopy of wing discs expressing Hh-GFP. Discs were labelled ex vivo with a rabbit anti-GFP antibody and then fixed and processed for cryosectioning. Ultra-thin sections, cut orthogonally to the V/D axis, were incubated with a fluorescent (Alexa594) 1.4-nm nanogold-conjugated anti-rabbit Fab’ probe. Labelled cryosections were first imaged at the fluorescence microscope ( a ) and then at the transmission electron microscope after silver enhancement of the nanogold signal ( b – p ). At the light microscopy level ( a ) fluorescent labelling is detected at apical areas and at basolateral regions of the P compartment. At the EM level, apical immunogold labelling ( c and d shows the area delimited by a red box in b ) decorated microvilli membranes (arrows in d ), whereas basolateral signal ( f – i shows EM images of the area delimited by a blue box in b , while j – p shows details of a different disc) is mainly associated with discrete extents of the plasma membrane (arrows in f , i , j ) that frequently coincide with cell-to-cell contacts (arrows in j ). Also, immunogold labelling is detected in clusters of EV-like structures (arrowheads in g,i,k,m,n,p), some of which are associated with cell protrusions (insets in f (g) and l ( m )). A and P compartments as well as apical (Ap) and basolateral (Bs) regions are indicated in a and b . To help the interpretation, apical and basolateral extracellular spaces are depicted in red ( c ) and blue ( f , i – p ), respectively. a to i correspond to the same wing disc, whereas j to p correspond to a different specimen. LD, lipid droplet. Scale bars, 25 μm ( a , b ), 5 μm ( e ), 500 nm ( c , h , j , l , o ), 200 nm (d,f,i ,k,m,n ) and 100 nm ( g,p ). Full size image Due to the size of some of these EVs (30–150 nm) and their association with MVBs, they could comprise bona fide exosomes [13] , defined as EVs enriched in cholesterol, sphingomyelin, ceramide and components of membrane raft microdomains [14] . Exosomes originate from MVBs and are released to the extracellular space following fusion with the plasma membrane, containing proteins implicated in trafficking, membrane fusion and signalling [15] . Hh has been shown to traffic from apical to basolateral plasma membranes [6] , [7] , [8] and this recycling process might actually localize Hh in MVBs. Both processes, Hh release [8] and MVB formation, require Rab5, Rab4 and Rab8 function [16] , [17] . Hh-loaded exovesicles in culture cells Further characterization using Drosophila cultured wing disc cells, Cl8, as well as transfected S2 cells expressing Hh-GFP also show the presence of endogenous Hh or Hh-GFP in EVs. These EVs have exosome-like features based on flotation density and protein markers ( Fig. 5 and Supplementary Fig. 2A,B ). Characterization of the vesicular fraction by isopynic density gradients shows co-fractioning of the Hh protein with membrane (TSG101, Rab11, Rab8 and Syntaxin), and luminal (Hsp70) exosomal-associated proteins [18] ( Fig. 5b ) and the Hh co-receptor Ihog ( Supplementary Fig. 2C ). Previously, it has been described that Hh is associated to lipoproteins ( Drosophila apoliproteins; Lipophorins (Lp-I and Lp-II [19] ) for transport [12] . Lp-II has also been detected in EV preparations in the presence of fly extracts (source of Lps in the Drosophila cell culture medium) but Lp-II does not co-fractionate with Hh-containing exosomes ( Fig. 5a,b ). Moreover, Hh-loaded EVs were able to activate the Ptc::luciferase reporter ( Fig. 5c,d ), further showing that the Hh protein present in these EVs is functional. 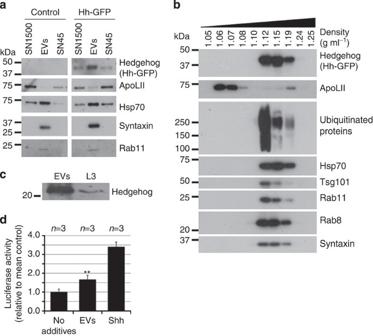Figure 5: Hedgehog protein is associated to EVs with features of exosomes. (a) A representative western blotting of supernatants (SN1500 and SN45) and EVs obtained from 5 ml of media from mock- (control) or Hh-GFP-transfected Cl8 cells. Similar volume of supernatants (1/350 of the total) and 1/5th of the EVs were applied to the gel. Antibodies against indicated proteins were used as described in Methods. Antibody against Hh showed that Hh is found in EVs, although the Hh-associated to EVs represents less than 10% of the total secreted forms (n=3). (b) EVs from Hh-GFP-transfected cells were fractionated by continuous sucrose density gradient and equal amounts (1/5th) of the resulting fractions analysed by western blotting. Specific antibodies show the presence of Hh and protein markers of exosomes (Ubiquitinated proteins, Hsp70, TSG101 and Rab11) mapping at similar densities. ApoLII was also tested in the gradient, showing a different pattern along the gradient. (c) Western blot analysis of Hh protein in EVs obtained from untransfected Cl8 cells and extract from larvae stage 3 (L3). (d) Luciferase activity in Cl8 cells transfected with ptcΔ136-GL3 Firefly responsible reporter and incubated without (Control) or with EVs obtained from Cl8 cells. Shh recombinant protein was used as positive inducer. Mean±s.d. of three replicates is shown. Significance level (Student’st-test) **P<0.01. Figure 5: Hedgehog protein is associated to EVs with features of exosomes. ( a ) A representative western blotting of supernatants (SN1500 and SN45) and EVs obtained from 5 ml of media from mock- (control) or Hh-GFP-transfected Cl8 cells. Similar volume of supernatants (1/350 of the total) and 1/5th of the EVs were applied to the gel. Antibodies against indicated proteins were used as described in Methods. Antibody against Hh showed that Hh is found in EVs, although the Hh-associated to EVs represents less than 10% of the total secreted forms ( n =3). ( b ) EVs from Hh-GFP-transfected cells were fractionated by continuous sucrose density gradient and equal amounts (1/5th) of the resulting fractions analysed by western blotting. Specific antibodies show the presence of Hh and protein markers of exosomes (Ubiquitinated proteins, Hsp70, TSG101 and Rab11) mapping at similar densities. ApoLII was also tested in the gradient, showing a different pattern along the gradient. ( c ) Western blot analysis of Hh protein in EVs obtained from untransfected Cl8 cells and extract from larvae stage 3 (L3). ( d ) Luciferase activity in Cl8 cells transfected with ptcΔ136-GL3 Firefly responsible reporter and incubated without (Control) or with EVs obtained from Cl8 cells. Shh recombinant protein was used as positive inducer. Mean±s.d. of three replicates is shown. Significance level (Student’s t -test) ** P <0.01. Full size image Finally, interfering with proteins involved in the production/secretion of EVs, TSG101 and Rab27 (refs 20 , 21 , 22 ) in Drosophila wing disc cells (Cl8 cells) leads to a significant reduction in the levels of Hh protein associated to EVs ( Supplementary Fig. 2D ). However, in our in vitro model, interference with the ESCRT-independent exosome production protein nSMase does not show a significant decrease in the Hh levels within EVs ( Supplementary Fig. 2D ). Together, the results obtained from cell cultured EV analysis support the notion that at least a fraction of functional Hh is secreted in exosome-like vesicles in Drosophila cells. Exovesicle formation genes are needed for Hh release in vivo From an in vivo perspective, preliminary observations have shown a reduction of the Hh gradient when blocking EVs formation via RNA interference (RNAi) treatment [6] . Further, in vivo RNAi screening confirmed the previously observed role of genes involved in EV formation and release, identifying new proteins involved in the graded secretion of Hh via EVs. Five RNAi treatments show an effect on the Hh gradient by the analysis of the Ptc::GFP-Enhancer-Trap expression, a recognized reporter for both, short- and long-range Hh responses: the ESCRT complex components Vps22 (ESCRT-II component) and Vps24 (ESCRT-III component), the ESCRT-independent sorting protein SMase [23] , the SNARE complex component Ykt6 and the Drosophila homologous for the P4-ATPase (CG31729), TAT-5 in C. elegans shown to regulate the budding of EVs from the plasma membrane (shedding vesicles/ectosomes/microparticles) [24] ( Fig. 6a–d ). All these proteins are involved in EV secretion pathways and Ykt6 has also been shown to be involved in the release of exosomes containing Wingless (Wg) [25] . 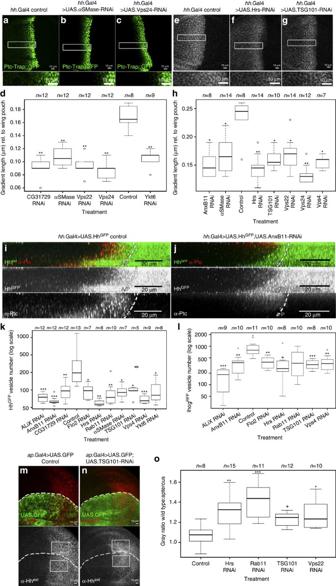Figure 6: Hh signalling and release in mutant conditions for exosome production genes. (a–h) Hh signalling in wing discs expressing RNAi treatments in the P compartment (b–d,f–h) and control (a,e), visualized in the A compartment using the Ptc-promotor-Trap::GFP reporter (a–d) and immunolabelling for the long-range target Ci (e–h). Detail shown at the bottom and anterior is to the left. Note in RNAi wing discs (b–d,f–h), gradients are shorter than in controls (a,e). (d,h) Box plot comparing gradient length expressed as a proportion of wing pouch length, between control discs and treatments for each reporter. (i–l) Quantification of the number of Hh-GFP (i–k) or Ihog-RFP (l) released punctate structures. Reconstruction inZ(lateral view) of wing discs expressing Hh-GFP (i) or co-expressing Hh-GFP and RNAi for AnxB11 (j) under the control ofhh.Gal4 and immunostained for the transcription target Ptc (red, also a marker of the A compartment cells), note punctate structures in the A compartment, decrease after RNAi treatment. (k) Boxplot comparing the number of Hh-GFP puncta released for the control (UAS.Hh-GFP) and 10 exosome-related treatments. Note the reduction in the number of puncta. (l) Boxplot comparing the number of Ihog-RFP puncta (anterior compartment) for the control (UAS.Ihog-RFP) and seven treatments related to exosome production. Note the reduction in the number of puncta. (m–o) Endogenous externalized Hh levels decrease in mutant conditions for exosome production genes.Ex vivostaining for Hh in wild-type discs (m) or in wing disc expressing RNAi for TSG101 (n) driven byap.Gal4 with a dorsal expression domain (marked by GFP), leaving the ventral domain in wild-type conditions as an internal control. Note the decrease in fluorescence after treatment (m,n). (o) Boxplot showing the ratio between relative intensity of the mean grey value in the dorsal (RNAi treated) versus the ventral compartment (wild type). The ratio is close to 1 in control, while the ratio for all RNAi cases is greater than 1 due to a decrease in the levels of external Hh in treated cells. Significance levels for pairwise tests (Tukey HSD or Wilcoxon, depending on Normality of data): ***P<0.001, **P<0.01, *P<0.05,+P<0.1. Scale bars,10 μm. In addition, to confirm the requirement of EV formation during Hh signalling, we have quantified the effect of knocking down a fraction of the genes identified over the long-range target Cubitus interruptus (Ci), and a significant decrease in activation was also observed ( Fig 6A,e–h ). These experiments then endorse the necessity of the molecular machinery for EV formation and release for both short- as well as long-range Hh signalling. Figure 6: Hh signalling and release in mutant conditions for exosome production genes. ( a – h ) Hh signalling in wing discs expressing RNAi treatments in the P compartment ( b – d , f – h ) and control ( a , e ), visualized in the A compartment using the Ptc-promotor-Trap::GFP reporter ( a – d ) and immunolabelling for the long-range target Ci ( e – h ). Detail shown at the bottom and anterior is to the left. Note in RNAi wing discs ( b – d , f – h ), gradients are shorter than in controls ( a , e ). ( d , h ) Box plot comparing gradient length expressed as a proportion of wing pouch length, between control discs and treatments for each reporter. ( i – l ) Quantification of the number of Hh-GFP ( i – k ) or Ihog-RFP ( l ) released punctate structures. Reconstruction in Z (lateral view) of wing discs expressing Hh-GFP ( i ) or co-expressing Hh-GFP and RNAi for AnxB11 ( j ) under the control of hh. Gal4 and immunostained for the transcription target Ptc (red, also a marker of the A compartment cells), note punctate structures in the A compartment, decrease after RNAi treatment. ( k ) Boxplot comparing the number of Hh-GFP puncta released for the control (UAS.Hh-GFP) and 10 exosome-related treatments. Note the reduction in the number of puncta. ( l ) Boxplot comparing the number of Ihog-RFP puncta (anterior compartment) for the control (UAS.Ihog-RFP) and seven treatments related to exosome production. Note the reduction in the number of puncta. ( m – o ) Endogenous externalized Hh levels decrease in mutant conditions for exosome production genes. Ex vivo staining for Hh in wild-type discs ( m ) or in wing disc expressing RNAi for TSG101 ( n ) driven by ap. Gal4 with a dorsal expression domain (marked by GFP), leaving the ventral domain in wild-type conditions as an internal control. Note the decrease in fluorescence after treatment ( m , n ). ( o ) Boxplot showing the ratio between relative intensity of the mean grey value in the dorsal (RNAi treated) versus the ventral compartment (wild type). The ratio is close to 1 in control, while the ratio for all RNAi cases is greater than 1 due to a decrease in the levels of external Hh in treated cells. Significance levels for pairwise tests (Tukey HSD or Wilcoxon, depending on Normality of data): *** P <0.001, ** P <0.01, * P <0.05,+ P <0.1. Scale bars,10 μm. Full size image To further analyse the effect of knocking down EVs production genes over Hh-loaded EVs in vivo , we ectopically expressed Hh-GFP or Ihog-RFP in producing cells, quantifying the visible punctate structures only in the A compartment ( Fig. 6i–l and for methods Supplementary Fig. 3 ). We tested RNAi treatments with a clear effect in Hh signalling ( Fig. 6a–h and ref. 6 ) including the ESCRT-0 protein Hrs [26] , the accessory ESCRT protein ALiX [26] , the EV component Anx B11 (ref. 27 ), the endosomal sorting protein Rab11 implicated in EV targeting [28] and the lipid raft component Flo2 also found in EVs [29] . All RNAi treatments tested result in significantly fewer Hh-GFP puncta in the A compartment ( Fig. 6i–k ), showing an effect on actual Hh secretion. Similar reduction effects were also observed for Ihog-RFP puncta, confirming again the role of these genes in the regulation of the Hh pathway ( Fig. 6k ). Moreover, interfering with EV production decreases the externalized levels of endogenous Hh (see Fig 6C,c expressed in levels of ratio change), shown by e x vivo staining after depletion only in the dorsal compartment of the disc, while the ventral part retains the wild-type conditions ( Fig. 6m,n ). Importantly, all RNAis used did not have a significant apoptotic effect after treatment ( Supplementary Fig. 4A ). In addition, quantitative reverse transcription-PCR (RT–PCR) experiments for four of these treatments confirmed the significant reduction of targeted RNA levels induced by the RNAis expression ( Supplementary Fig. 4B ). On the other hand, immunolabelling for total endogenous Hh levels of wing discs expressing the RNAi constructs only in the dorsal compartment, and compared to the wild-type ventral compartment, show no significant change, excluding potential effects of RNAi treatments over production or degradation of intracellular Hh ( Supplementary Fig. 4C ). The only exceptions to the latter observation were the RNAi treatment for the ESCRT-I component TSG101 and the ESCRT-II component Vps22, which show significant accumulation of total Hh on the P compartment (paired t -test, t =−5.19, df=7, P <0.01; Supplementary Fig. 4C,c ). However, despite this accumulation, both TSG101 and Vps22 RNAi treatment still lead to a reduction in the extracellular levels of Hh ( Fig. 6m–o ). Thus, taking into account all data from RNAi treatments, EV production is required for the normal release levels of Hh to the extracellular space in the wing disc and consequently for the normal graded signalling pattern. Our previous research showed a requirement for cytonemes extending from Hh producer cells towards receptor cells for Hh gradient formation, while Hh was also observed in punctate structures [6] . Here we characterized these puncta confirming their EV nature and role during Hh signalling. These Hh-loaded exovesicles are a heterogeneous group, differing in size and potentially in origin. In vivo imaging shows puncta moving along cytonemes, suggesting a route of Hh secretion and restricted dispersion where Hh-containing EVs are transported by cytonemes. Nevertheless, to date, we still do not know the precise mechanism used for Hh release and transport along the cytoneme. Ultrastructural analysis confirmed the presence of Hh in MVBs on the A compartment, supporting an ESCRT dependent route of exovesicle formation and release. Thus, it is possible that MVBs fuse to the plasma membrane-releasing vesicles at the same time as cytonemes are elongating. Alternatively or in addition, smaller vesicles (that may well be small MVBs) appear to be travelling within the cytoneme. However, live imaging of these structures also shows puncta shedding directly from the cytonemes, and these might correspond to membrane-derived vesicles known as shedding vesicles or ectosomes/microvesicles [30] . Ectosome EVs were described as bigger than exosomes and more heterogeneous in size, ranging from 200 nm to greater than 1 μm in diameter, and are originated by shedding preceded by the budding of small cytoplasmic protrusions, which then detach by fission of their stalk [30] . Although shedding vesicles/ectosomes seem to have a different origin [31] , the mechanisms of their sorting process remain obscure and might also be dependent on the ESCRT complex [24] . In addition, studies have shown a crucial role for cholesterol-rich microdomains of the plasma membrane for shedding vesicle formation [32] as well as for biogenesis of exosomes [14] . In our in vivo experiments, we have observed a decrease in Hh signalling by knocking down Vps22, an ESCRT-II complex component described as dispensable for vesicles derived directly from the plasma membrane [33] , [34] , but required for MVB formation [35] (reviewed in ref. 36 ) supporting an MVB fusion origin. However, we have also observed a decrease in signalling and Hh release when interfering with P4-ATPase (CG31729), the Drosophila orthologue of TAT-5 specifically involved in the formation of ectosomes in C. elegans [24] . Thus, as it is difficult to account for the considerable differences between the two types of vesicles, the result of knocking down Vps22 and P4-ATPase together with the EM data and the in vivo imaging indicate that Hh might be released in both ectosomes/microvesicles and exosome-like vesicles. Determining which process might be the main one regulating Hh secretion or whether both processes are linked is a future challenge. In vitro , functional tests demonstrate that Hh-loaded exovesicles fractionate together with classical exosomal markers ( Fig. 5b ), and are able to activate Hh-dependent transcription in cell culture ( Fig. 5d ). Furthermore, interference with genes involved in the formation and release of EVs in vivo has a decreasing effect on the release of Hh to the extracellular space, altering the Hh gradient formation during signalling ( Fig. 6 ). In our experimental model (the Drosophila wing imaginal disc), all RNAi treatments behave similarly, independent of their individual function within the EVs formation pathways. The only exceptions were given by the silencing of ESCRT-I component TSG101 and the ECRT-II component Vps22, which resulted in a significant accumulation of total Hh in the P compartment ( Supplementary Fig. 4C ) but still impaired Hh secretion to the A compartment ( Fig. 6i–o ), probably due to a simultaneous impairment of the route for Hh degradation as they both play a key role in MVB formation [26] , [35] . Differential outputs after downregulation of different EVs formation genes have been reported, including an increment in EVs release (for example, ALiX RNAi) [26] . However, there is an increasing evidence of the heterogeneous nature of EVs in size, protein content and origin [18] . Depletion of a gene involved in the formation pathway might either affect EVs release in general or might alter the proportion of the different vesicles formed [26] . Thus, quantifying the effects over those vesicles containing Hh or Ihog might not detect potentially distinct changes in the distribution of different size vesicles or protein content. Association of Hh to EVs, and thus membranes, supports the transport mechanism initially proposed by Greco et al. [37] for the spread of Wg protein; Wg secreted and moved while contained in membrane fragments called argosomes. Vesicular release of SHh has also been described in the determination of left–right asymmetry in vertebrates [38] . Moreover, Hh has been found in exosomal structures for its apical secretion in C. elegans [39] . We have found a functional Hh associated to heterogeneous EVs, either originated from MVBs or/and directly shedding from the plasma membrane of cytonemes, and that are essential for Hh gradient formation. Recent reports also show Wg and Wnt to be released in exosomes at the wing disc, in the zebrafish and tissue culture cells [21] , [22] , [25] , [40] . During patterning of the zebrafish neuroectoderm, Wnt8a localizes to the membrane-associated punctate structures in live tissue and these puncta are found on filopodial cellular processes [40] . In Drosophila , Wg has also been visualized in vivo moving along cellular extensions by Evi-exosomes [18] or released as exosomes from MVBs at synaptic terminals [22] . The release of exosomes and further activation of the Hh pathway in an epithelium might then require a synaptic process with a potential complex association of various proteins. Thus, in vitro experiments with cultured cells might not be able to reproduce the signalling process in an epithelium, leading to the relatively low representation of Hh in exosomes and Hh-dependent transcription activation. Overall, our results support a route for morphogen transport that involves vesicle transport and secretion along cytonemes to accomplish proper spatially restricted signalling. Still, key unanswered questions regarding the final transfer or release of morphogens like Hh remain. Supporting a conserved mechanism in vertebrates, SHh and CDO (vertebrate homologue of Ihog) in vesicle-like structures have been observed moving along specialized filopodia in the chick limb bud [9] . Further elucidation of the origin, structure and function of the EVs implicated in this process as well as the mechanism of their release is likely to be essential to understand Hh cell-cell signalling. However, our results do not totally exclude a potential combinatorial effort with other secretion routes or extracellular forms of Hh, such as lipoprotein particles [12] , [41] or Hh multimers [42] . Comprehending how signalling molecules like Hh are distributed will improve the knowledge of developmental processes and their role in diseases like cancer, revealing a wider set of mechanisms and genes involved in the regulation of their signalling. Fly mutants A description of mutations, insertions and transgenes ( Supplementary Table 1 ) is available at Fly Base ( http://flybase.org/ ). Gal80 ts , FLP122 (Bloomington Drosophila Stock Centre (BDSC), Indiana, USA; http://flystocks.bio.indiana.edu ). Overexpression experiments Gal4 drivers were: hh. Gal4 (ref. 43 ), ap. Gal4 (ref. 44 ), tub .Gal4 (BDSC). The pUAS-transgenes were: UAS.Hh-GFP [45] , UAS.Ihog-RFP, UAS.Ihog-YFP, UAS.Ihog-CFP [7] , [8] , UAS.CD63-GFP [12] , UAS.CD4-tdTom [46] and UAS.eGFP (BDSC). UAS-RNAi lines targeting TSG101 (35710), ALiX (33417), Hrs (33900), Rab27 (37774), Vps 22 (38289), Vps 24 (38281), αSmase (25283) and Ykt6 (38314) were from BDSC. Flo2 (31525), AnxB11 (29693), Rab11 (108382), P4-ATPase (CG31729) (105987) and Vps4 (105977) were from the IMP Vienna Drosophila RNAi Centre (VDRC; http://stockcenter.vdrc.at ). Transient expression of UAS constructs using Gal4; TubGal80 ts drivers was achieved by maintaining fly crosses at 18 °C and inactivating Gal80 ts at the restrictive temperature (29 °C) for thirty hours before dissection. Immunostaining of imaginal discs Immunostaining was performed according to standard protocols [47] , [48] . Imaginal discs from third instar larvae were fixed in 4% paraformaldehyde (PFA)/PBS for 20 min at room temperature (RT) and washed in PBT before incubating with PBT 0.2% bovine serum albumin for blocking (1 h at RT) and primary antibody incubations (overnight at 4 °C). Incubation with fluorescent secondary antibodies (1/200 Jackson laboratories and Invitrogen, Carlsbad, CA) was performed for 2 h at RT for posterior washing and mounting in media (Vectashield). Antibody dilutions were: rabbit polyclonal anti-Hh (1:800 or 1:500, raised in this work); rat monoclonal anti-Ci [48] (1:20 dilution, a gift from B. Holmgren); rabbit polyclonal anti-GFP antibody (1:500, Molecular Probes, A-6455); and rabbit polyclonal anti-Caspase 3 antibody (1:50 dilution, Asp-175 from Cell Signalling). Ex vivo labelling using anti-GFP antibody is described in ref. 45 . Imaginal discs from third instar larvae were dissected on ice, transferred immediately to ice-cold M3 medium containing anti-Hh (1:30 dilution; rabbit antibody raised for this work), anti-GFP (1:50 dilution, rabbit antibody A-6455; Invitrogen) or anti-Disp [8] (1:50 dilution, guinea pig antibody), or anti-Dlp (1:5 dilution; mouse antibody, Hybridome bank, Iowa) antibodies and incubated at 4 °C for 30 min. The incubation with the primary antibody under these ‘ in vivo ’ conditions, without detergents before fixation rendered the antibody incapable of penetrating the cells. They were then washed in ice-cold PBS, fixed in PBS 4% PFA at 4 °C, washed in PBT and incubated with secondary fluorescent antibody as above. In vivo imaging of abdomen Pupae were filmed through a window in the pupal case for analysis [49] . The window was made with forceps after attaching the pupa to double-sided adhesive tape. To remove the adhesive, water was used. Mounting between two spacers made of five bands of Parafilm ‘M’ ensured minimal squashing. The pupa was surrounded by water, placing a coverslip over the sample and closing the open part of the chamber with voltalef oil to ensure oxygen supply. All imaged flies developed into pharate adults and many hatched. Z-stacks of around 40 μm with a step size of 2.5 or 3 μm were recorded every 150–180 s using a Leica SP8 confocal microscope at 24±1°C. [49] Number ( N ) of recorded pupae: Supplementary Movies 2 and 7 , N =8; Supplementary Movie 3 , N =3; Supplementary Movies 4 and 5 , N =9; Supplementary Movie 6 , N =6. Microscopy and image processing of imaginal discs Laser scanning confocal microscopes (LSM510 or LSM710 Vertical; Zeiss) were used for confocal fluorescence imaging of imaginal discs. ImageJ software (National Institutes of Health) was used for image processing and for determining fluorescence levels. Quantification of EVs and Hh levels Vesicle number ( Fig. 6i–l ) was quantified using ImageJ. A rectangular area of 170 × 75 μm was chosen and allocated in the A compartment in the vicinity of the P compartment ( Supplementary Fig. 3A,B ). The edge limit of the P compartment cells was defined by creating a shaped selection after blurring of the projected image ( Supplementary Fig. 3A,B ); also confirmed by the immunolabelling of the A compartment Ptc expression ( Supplementary Fig. 3C ). Within the selection a mean filter of one pixel radius was used to smooth the image and remove noise. To remove particles that were of low fluorescence intensity, the lower threshold for pixel intensities was set to 60, whereas the upper was kept at 255. Finally, the ‘Analyse Particles’ tool was used to count puncta within 0–4.5 pixels of size ( Supplementary Fig. 3A,B ). Quantifications were performed using individual Z slices taken every 1μm. All images were treated identically. For all RNAi treatments, a control for potential cell death due to RNAi treatment was performed by immune-staining with anti-Caspase antibody (see Supplementary Fig. 4A ); no significant increment of cell death due to treatment was detected. Levels of externalized Hh ( Fig. 6m–o ) and total Hh ( Supplementary Fig. 4C ) were quantified by determining Mean Grey Value in ImageJ. A rectangular area of approximately 14,400 pixels within the wing pouch on each side of the dorsoventral border marked by GFP expression driven by the ap. Gal4 was used. Quantification of gradient length Gradient lengths were determined as described in ref. 6 and expressed as a proportion of wing pouch length ( Fig. 6a–h ). Quantitative RT-qPCR The RNAis’ ability to downregulate target genes in transgenic flies was already tested by the manufacturer (BDSC Trip toolbox stocks). Four RNAi treatments were tested ( Supplementary Fig. 4B ). Three independent biological replicate assays were produced for TSG101-, Flo2-, Rab11- and control EGFP-RNAi constructs, and six replicates in the case of HRS- and its control EGFP-RNAi. For RNA extraction, Drosophila third instar larvae generally expressing RNAi constructs or not were collected and kept at −80 °C. Larval tissues were homogenized in 500 μl Trizol (Invitrogen), 100 μl Chloroform (Merck). After a 15 min 15,000 g centrifugation at 4 °C, the upper phase containing total RNA was collected and precipitated with 250 μl 2,3-propanol (Merck). The dry pellets were resuspended in 40 μl sterile water and stored at −80 °C. For RT-qPCR reaction, RNA concentration was measured using Nanodrop ND-1000 and RNA integrity was confirmed using the ‘Total RNA Analysis ng sensitivity (Eukaryote)’ assay of the Agilent 2100 bioanalyzer. cDNA was generated using Super Script III First-Strand Synthesis SuperMix for qRT–PCR from Invitrogen (PN 11752250), 800 ng of total RNA were used for each replicate in a final volume of 20 ul (final concentration of 40 ng μl −1 ). qPCR reactions (95 °C for 10 min., 40 cycles of 95 °C for 15 s and 60 °C for 30 s; and 1 cycle of 95 °C for 15 s, 60 °C for 15 s and 95 °C for 15 s) were run on the CFX 384 (Biorad) according to manufacturer's instructions. Primers are displayed in Supplementary Table 2 . Statistical analysis All statistical analysis was carried out in R [50] . Data were tested for normality using Shapiro–Wilk tests (data were logged for normality where required), and for homogeneity of variance using Bartlett tests. Models for treatment effects on gradient length For the Ptc reporter, a Kruskal–Wallis test of gradient length against treatments related to exovesicle production (wild type, UAS-aSmase-RNAi , UAS-Vps22-RNAi , UAS- Vps24-RNAi , UAS-Ykt6-RNAi , UAS-CG31729 (P4-ATPase)-RNAi ) ( n =65) showed a significant treatment effect ( χ 2 -test [2] =34.11, df=5, P <0.001). For the Ci reporter, a Kruskal–Wallis test of gradient length against treatments related to exovesicle production (wild type, UAS-Hrs-RNAi , UAS-Vps22-RNAi , UAS- Vps4-RNAi, UAS-Anxb11-RNAi, UAS-TSG101-RNAi, UAS-Vps24-RNAi, UAS- α Smase-RNAi ), ( n =87) showed a significant treatment effect ( χ 2 =36.89, df=7, P <0.001). Pairwise Wilcoxon tests adjusted for multiple comparisons were used to test for differences between control and each treatment ( Fig. 6d,h ). Models for treatment effects on number of EVs released A Kruskal–Wallis test of the number of Hh-GFP puncta released for control (UAS-Hh-GFP) and 10 EV-related treatments (UAS-ALIX-RNAi, UAS-AnxB11-RNAi, UAS-CG31729 (P4-ATPase)-RNAi, UAS-Rab11-RNAi, UAS-Hrs-RNAi, UAS-Vps4-RNAi, UAS-Flo2-RNAi, UAS-TSG10-RNAi, UAS-YKT6-RNAi and UAS-aSmase-RNAi)( n =103) showed a significant treatment effect ( χ 2 =54.67, df=10, P <0.001). A Kruskal–Wallis test carried out for the number of Ihog-RFP puncta released for control ( UAS-Ihog-RFP ) and seven treatments related to exosome production ( UAS-Alix-RNAi , UAS-TSG101-RNAi , UAS-AnxB11-RNAi , UAS-Rab11-RNAi , UAS-Hrs-RNAi , UAS-Vps4-RNAi , UAS-Flo2-RNAi) ( n =76) showed a significant treatment effect ( χ 2 =31.18, df=7, P <0.001). Pairwise Wilcoxon tests adjusted for multiple comparisons were used to test for significant differences between control and each treatment ( Fig. 6k,l ). Models for treatment effect on endogenous levels of external Hh A paired t -test comparing relative fluorescence (mean grey values) for wild-type tissue and RNAi-treated tissue ( UAS-TSG101-RNAi , UAS-Rab11-RNAi , UAS-Hrs-RNAi , UAS-Vps22-RNAi ) ( n =56) showed a significant difference ( t =13.18, df=55, P <0.001). The Ratio WT: ap was tested for difference between RNAi expressing wing discs ( ap ) and discs without RNAi treatment or Control (WT), using Anova (F 4,51 =7.79, P <0.001). Tukey’s Honest significant difference tests were used to test for differences between control and each treatment ( Fig 6c,e ). Models for treatment effect on endogenous levels of total Hh Paired t -tests comparing the relative fluorescence (mean grey values) for wild-type tissue and RNAi-treated tissue ( UAS-TSG101-RNAi , UAS-Hrs-RNAi , UAS-AnxB11-RNAi , UAS-Flo2-RNAi , UAS-Vps22-RNAi and UAS-CG31729-RNAi (P4-ATPase ) ( n =49) showed non-significant differences, except for TSG101 ( t =−5.19, df=7, P <0.01) and Vps22 ( t =−5.50, df=7, P <0.001) treatments. The Ratio WT: ap was tested for difference between RNAi expressing wing discs ( ap ) and discs without RNAi treatment or control (WT), using analysis of variance (F 6,42 =11.7, P <0.001). Tukey’s Honest significant difference tests showed that the only significant differences with control were for TSG101 ( P <0.05) and Vps22 ( P <0.001; Supplementary Fig. 4C,c ). Models for treatment effects on target RNA levels Welch two sample t -tests comparing the normalized values for RNA expression for wild-type tissue and each RNAi-treated tissue ( UAS-TSG101-RNAi , UAS-Flo2-RNAi , UAS-Rab11-RNAi , UAS-Hrs-RNAi ) showed significant differences between RNAi expressing larvae and larvae without RNAi treatment or Control ( Supplementary Fig. 4B ). Values for each treatment are: TSG101 RNAi against Control ( n =6; t =3.63, df=3.6, P <0.05), Flo2 RNAi against Control ( n =6; t =9.19, df=2.5, P <0.005), Rab11 RNAi against Control ( n =6; t =18.2, df=2, P <0.005), HRS RNAi against Control ( n =12; t =4.08, df=8.3, P <0.005). Immunoelectron microscopy Larvae were inverted in PBS and fixed in 2% (w/v) PFA and 0.2% (w/v) glutaraldehyde or 4% PFA and 0.05% glutaraldehyde in 0.1 M phosphate buffer (PB, pH 7.4) for 2 h at room temperature and kept in 1% (w/v) PFA in PB at 4 °C. Subsequently, wing discs were dissected, embedded in 10% (w/v) gelatine and processed for cryosectioning. Discs were cut orthogonal to the ventral/dorsal axis on an EM FCS cryo-ultramicrotome (Leica Microsystems) at −120 °C. For immunogold labelling, thawed 90-nm thick cryosections were incubated with rabbit anti-GFP (1:500, A-6455; Invitrogen, rabbit anti-Hh (1:150) (6), guinea pig anti-Disp (1:100) antibodies followed by protein A conjugated to 15-nm gold particles (EM Laboratory, Utrecht University, The Netherlands). Sections were stained with a mix of 1.8% methylcellulose and 0.4% uranyl acetate. For double labelling, anti-Disp [8] and anti-Hh [48] antibodies were detected with goat anti-guinea pig IgG conjugated to 10-nm gold particles and goat anti-rabbit IgG conjugated to 15-nm gold particles (British Biocell), respectively. For ex vivo anti-GFP labelling experiments, discs expressing Hh-GFP were labelled with 1:30 dilution anti-rabbit anti-GFP polyclonal antibody (Life technologies (Molecular Probes)) as above and reported in ref. 45 and fixed with 4% PFA and 0.05% GL in 0.1 M PB (pH 7.4) for 2 h at RT. The discs were processed for cryosectioning as described. Ultra-thin (100 nm) thawed cryosections were incubated with an anti-rabbit Fab′ fragment conjugated to Alexa594 and 1.4-nm nanogold (Fluoronanogold, Nanoprobes, New York, USA), mounted with 50% glycerol and visualized with an inverted fluorescence microscope (DMI6000, Leica Microsystems, Wetzlar, Germany). For EM visualization, nanogold labelling was amplified by silver enhancement according to manufacturer’s instructions (Nanoprobes). Sections were stained with a mixture of methylcellulose and uranyl acetate and visualized with a JEOL JEM 1010 (Tokyo, Japan) electron microscope at 80 kV. Images were recorded with a 4 × 4 k CMOS F416 camera from TVIPS (Gauting, Germany). Immunoprecipitation We modified a standard protocol for immunoprecipitation using Drosophila embryos [51] . Larvae expressing CD63-GFP, Ihog-RFP or co-expressing both under tub .Gal4 were collected and dry frozen in liquid Nitrogen. Fifty frozen larvae for each genotype were homogenized in 1 ml each of C Buffer (50 mM HEPES (pH 7.4), 50 mM KCl, 1 mM MgCl, 1 mM EGTA, 0.1% Triton, Protease inhibitors cocktail (Roche) and 1 mM PMSF). Extracts were initially clarified by centrifugation at 35,000 g for 10 min, followed by two high-speed centrifugations at 35,000 r.p.m. for 10 and 30 min. The supernatant was incubated with GFP-Trap coupled to agarose beads (Chromoteck) for 1 h at 4 °C, then washed (5 × ) with C Buffer. Immunoprecipitated samples were resuspended in sample buffer with DTT and subjected to 1 D SDS-polyacrylamide gel electrophoresis and western blotting. Blotted membranes were probed with appropriate antibodies, either to RFP (1:5,000, Abcam) or GFP (1:1,000, Sigma). After antibody stripping (Tris–HCL 0.5 M, pH 6.8, 2% SDS and β-mercaptoethanol 0.1 M, for 30 min at 60 °C) membranes were probed with anti-Hh (rabbit antibody raised for this work 1:5,000). Uncropped western blots are shown in Supplementary Fig. 5A–C . Cell culture Drosophila S2 cells stably-expressing full-length Hh fused to GFP (S2::Hh-GFP) were generated using multicistronic vector pAc5-STABLE2-Neo [52] , and cultured in Schneider’s medium supplemented with 10% fetal bovine serum (FBS) and 1% penicillin/streptomycin at 25 °C. Cl8 cells were cultured in M3 medium containing 2.5% of FBS, 2.5% fly extract, 10 mg ml −1 of insulin and 1% penicillin/streptomycin. Transient transfections of Cl8 cells were performed using X-tremeGENE transfection reagent (Roche Applied Science) following manufacturer’s instructions on 25 million (5 million ml −1 ) cells and 6 μg of DNA per transfection experiment. Production and isolation of EVs Crude preparation of EVs from Hh-GFP transiently transfected Cl8 cells was obtained by collecting 5 ml of EV-depleted media and performing differential centrifugation at 2,000 g and 100,000 g of supernatants after 48 h transfection. Pellets containing crude EVs were resuspended. For EV production of S2::Hh-GFP and Cl8 cells, 400 million cells were cultured for 48 and 96 h, respectively, in EV-depleted media (2.5 millions ml −1 ) and exosomes-enriched EVs secreted into the medium were purified as previously described [53] ; briefly, culture supernatant was collected and centrifuged at 2,000 g , 4 °C, for 10 min to remove cells. The resultant supernatant was subjected to filtration through 0.22-μm pore filters, followed by ultracentrifugation at 10,000 and 100,000 g for 30 and 60 min, 4 °C, respectively. Resulting pellets were washed with PBS and again ultracentrifuged at 100,000 g , 4 °C, for 60 min. Final pellets were suspended in PBS and stored at −80 °C. Western blot analysis A small portion (1/350th) of supernatants obtained after 2,000 and 100,000 g , and 1/5th of the crude EVs preparations or the fractions from the sucrose gradient were analysed by western blotting. Extracts from larvae stage 3 (L3) were prepared as described [7] . SDS sample buffer was added to samples and incubated for 5 min at 37, 65 and 95 °C and separated on 4–12% pre-casted acrylamide gels (Invitrogen) under non-reducing conditions. Gels were transferred to polyvinylidene difluoride membranes and blocked (5% milk and 0.05% Tween-20 in PBS) for antibody incubation. Chemoluminescent detection of proteins was performed using ECL Prime (Amersham) or Clarity Western ECL substrate (Biorad). Monoclonal antibodies were purchased from vendors indicated: anti-GFP (clones 7.1 and 13.1) from Roche, anti-GFP (clone GFP-20) for co-immunoprecipitation experiments from Sigma, anti-RFP (ab62341) from Abcam, anti-Hsp70 (BRM-22) from Santa Cruz Biotechnology, Inc (Santa Cruz, CA), anti-TSG101 (4A10) from Abcam, anti-Rab11 (clone 47) and anti-ubiquitin (clone 6C1.17) from BD Biosciences (Mountain View, CA), anti-ApoLII (ref. 54 ) and anti-Syntaxin (8C3) from Developmental Studies Hybridoma Bank (Iowa City, IA). Rabbit polyclonal anti-Hh and anti-Ihog were obtained using the Polyclonal Genomic Antibody TechnologyTM (sdix) [55] . For anti-Hh production, the immunogen region used comprised the DmHh amino-acids region 80–256; as for the anti-Ihog the DmIhog amino-acid region 248–488 was used. Horseradish peroxidase-conjugated secondary antibody was from GE-Healthcare (Buckinghamshire, UK). Uncropped Western blots are shown in Supplementary Fig. 5 . Fractionation of EVs on continuous sucrose gradient A continuous 0.25–2 M sucrose gradient in 20 mM HEPES (pH 7.4) was performed as described in ref. 56 . Briefly, EVs were placed on the continuous sucrose gradient and submitted to ultracentrifugation for 16 h at 210,000 g , 4 °C, in a SW40Ti swinging-bucket rotor. By using an auto densi-flow density gradient fractionator (Labconco, Kansas City, MO, USA), 1 ml fractions were collected from top to bottom and 20 μl of each fraction were reserved for measurement of the refractive index to density determination. Each fraction was diluted with 2 ml of 20 mM HEPES (pH 7.4) and ultracentrifuged for 1 h at 100,000 g , 4 °C, in a TLA-110 rotor. Supernatants were aspirated and pellets were suspended in 25 μl PBS and stored at −80 °C. Gene silencing in Drosophila cultured Cl8 cells nSMase, TSG101 and Rab27 dsRNAs were synthesized following the protocol used at the Drosophila RNAi Screening Centre (DRSC) in Boston. Briefly, DNA templates containing T7 promoters sequence on both ends were obtained from DRSC and were amplified by PCR. These PCR products were used for in vitro transcription reaction, which was carried out for 16 h at 37 °C using the T7 Megascript kit from Ambion. After DNaseI (Ambion) digestion to remove the template DNA, dsRNAs were purified using RNAeasy columns (Qiagen). Both PCR-amplified DNA and purified dsRNA products were assessed by gel electrophoreses and absorbance measurements of yield. Cl8 cells were seeded in six-well plates at 2 × 10 6 per well in 0.5 ml of FBS-free medium and 7.5 μg of dsRNA were added and incubated for 1 h, adding 1.5 ml of EV-depleted medium. After 48 h of incubation, a new dose of dsRNA was added and after another 48 h of incubation supernatants were collected and centrifuged at 2,000 g for 10 min to remove cells, then centrifuged at 100,000 g for 1 h, 4 °C, in a TLA-110 rotor. The resulting pellets were suspended in 25 μl of PBS and stored at −80 °C for subsequent analysis by western blotting. Luciferase activity assay of Hh EVs on cultured Drosophila cells Cl8 cells were transfected with ptcΔ136-GL3 Firefly responsible reporter [57] . After 24 h, cells were lifted and seeded into 96-wells plate, and 8-hours later incubated with 0.2 ng μl −1 of Shh recombinant protein (Sigma) or 1/4th of the crude EVs. After 24 h of treatment, Firefly luciferase levels were measured using Dual-Glo Luciferase Assay System (Promega) and the ratio to the control (no EVs added) was calculated to give Hh signalling activity. This was tested in triplicate and significant differences were tested by a t -student test. How to cite this article: Gradilla, A.-C. et al. Exosomes as Hedgehog carriers in cytoneme-mediated transport and secretion. Nat. Commun. 5:5649 doi: 10.1038/ncomms6649 (2014).